Unique S-scheme heterojunctions in self-assembled TiO2/CsPbBr3hybrids for CO2photoreduction Exploring photocatalysts to promote CO 2 photoreduction into solar fuels is of great significance. We develop TiO 2 /perovskite (CsPbBr 3 ) S-scheme heterojunctions synthesized by a facile electrostatic-driven self-assembling approach. Density functional theory calculation combined with experimental studies proves the electron transfer from CsPbBr 3 quantum dots (QDs) to TiO 2 , resulting in the construction of internal electric field (IEF) directing from CsPbBr 3 to TiO 2 upon hybridization. The IEF drives the photoexcited electrons in TiO 2 to CsPbBr 3 upon light irradiation as revealed by in-situ X-ray photoelectron spectroscopy analysis, suggesting the formation of an S-scheme heterojunction in the TiO 2 /CsPbBr 3 nanohybrids which greatly promotes the separation of electron-hole pairs to foster efficient CO 2 photoreduction. The hybrid nanofibers unveil a higher CO 2 -reduction rate (9.02 μmol g –1 h –1 ) comparing with pristine TiO 2 nanofibers (4.68 μmol g –1 h –1 ). Isotope ( 13 CO 2 ) tracer results confirm that the reduction products originate from CO 2 source. The depletion of fossil fuels and continuous CO 2 emissions have caused emerging global energy and environmental crises [1] , [2] , [3] , [4] , [5] . The photoreduction of CO 2 into renewable fuels with solar energy is recognized as a potential solution to solve above issues [6] , [7] , [8] , [9] , [10] . As a chemically inert, nontoxic and earth-abundant photocatalyst, TiO 2 is supposed to be proverbially utilized for CO 2 photoreduction [11] , [12] , [13] . However, like the majority of unitary photocatalysts, the photocatalytic efficiency of TiO 2 is still far away from the practical requirements largely due to its rapid electron–hole recombination [14] , [15] . Hybridizing TiO 2 with another semiconductor with a suitable band structure is a widely adopted strategy to tackle this issue owing to the efficient separation of photoinduced electron–hole pairs [16] , [17] , [18] , [19] , [20] . Therefore, it is of significance to explore or design a TiO 2 -based heterojunction to improve the photocatalytic CO 2 reduction performance. CsPbBr 3 , a typical material of halide perovskites, has attracted significant scientific interest in optoelectronic applications owing to its outstanding properties, including narrow photoemission, high photoluminescence quantum yield, tunable bandgap, and competing optoelectronic properties [21] , [22] , [23] , [24] . Inspired from the achievements in optoelectronic applications, CsPbBr 3 is a potential candidate for conducting efficient photocatalysis [25] , [26] . CsPbBr 3 quantum dots (QDs) have recently been hybridized with 2D graphene oxide [27] and porous g-C 3 N 4 [28] for CO 2 photoreduction. Nevertheless, in these cases, the electrons in the conduction band of CsPbBr 3 transferred into graphene and g-C 3 N 4 , forming Schottky and type-II heterojunctions, respectively, sacrificing the reduction ability of the photoinduced electrons despite achieving better charge separation. Very recently, an S-scheme heterojunction composed of two n-type semiconductors has been proposed [29] , [30] . The transfer path of photogenerated charge carriers at interfaces is like an “S” figure, enabling the heterojunctions to have the highest redox ability. The S-type charge transportation correlates with the band bending and internal electric field (IEF) at the junction. The n-type nature and remarkably different work functions of TiO 2 and CsPbBr 3 suggest a high possibility of forming S-scheme TiO 2 /CsPbBr 3 heterojunctions. Up to now, however, constructing perovskite CsPbBr 3 with TiO 2 , an emerging photoactive material and the most widespread photocatalyst, for efficient CO 2 photoreduction has not yet been reported. Herein, we report on a unique TiO 2 /CsPbBr 3 S-scheme heterojunction built by electrostatic self-assembly of TiO 2 nanofibers and CsPbBr 3 QDs for boosted photocatalytic CO 2 reduction. TiO 2 nanofibers show no aggregation upon dispersion in solution and thereby retain their phototactically active sites exposed on the surface. Meanwhile, randomly stacked TiO 2 nanofibres readily form a loose network, facilitating the adsorption–desorption and transportation of reactants and products. More importantly, the TiO 2 nanofibres are composed of small nanocrystals, possessing interparticle voids and rough surface, which make TiO 2 nanofibres an ideal host to anchor CsPbBr 3 QDs. Experimental study and density functional theory (DFT) calculation verify the presence of IEF in the unique TiO 2 /CsPbBr 3 heterojunction, which separate photoinduced charge carriers more efficiently. We argue the formation of the S-scheme charge transfer route at TiO 2 /CsPbBr 3 interfaces upon light irradiation. The obtained TiO 2 /CsPbBr 3 heterojunction shows a superior activity for reducing CO 2 into solar fuels under UV–visible-light irradiation. This work provides a point of view in TiO 2 -based photocatalyst for efficient CO 2 photoreduction driven by the S-scheme electron transfer route. Characterization of as-prepared CsPbBr 3 QDs Transmission electron microscopy (TEM) images with different magnifications are shown in Fig. 1a, b . The CsPbBr 3 QDs were of nanocubes with a size of 6–9 nm (inset in Fig. 1a ). High-resolution TEM (HRTEM) image (Fig. 1c ) showed lattice spacings of 0.413 nm, corresponding to the (110) facets of CsPbBr 3 . As-prepared CsPbBr 3 QDs were of cubic phase (JCPDS No. 54-0752) as revealed by X-ray diffraction (XRD) pattern (Fig. 1d ). The UV–vis absorption spectrum of CsPbBr 3 QDs revealed strong bands at 450 and 500 nm (Fig. 1e ). The corresponding photoluminescence (PL) spectrum unfolded a narrow emission at 520 nm, agreeing with previous reports [21] , [31] . Accordingly, the QDs solution showed a bright green fluorescence under 365 nm UV light (inset of Fig. 1e ). Fig. 1: Characterization of CsPbBr 3 QDs. a , b Transmission electron microscopy (TEM) image and corresponding size distribution (lower right inset of panel a ), the geometrical structure (upper right inset of panel a ), c high-resolution TEM (HRTEM) image, d X-ray diffraction (XRD) pattern, and e UV–vis absorption (black line) and PL emission (red line). Inset shows the photograph of CsPbBr 3 QDs colloidal solutions in hexane under UV light of 365 nm. Full size image Characterization of TiO 2 /CsPbBr 3 heterojunction The TiO 2 /CsPbBr 3 heterojunction was synthesized via electrostatic self-assembly of TiO 2 nanofibers and CsPbBr 3 QDs. Moreover, the minimization of the surface energy of the QDs should also be responsible for their adsorption to the TiO 2 nanofibers. The TiO 2 /CsPbBr 3 hybrids were denoted as TC x , where T and C denote TiO 2 and CsPbBr 3 QDs, respectively; x represents the weight percentage of CsPbBr 3 with respect to TiO 2 . The phase structures of TiO 2 , TC2, and TC4 were determined via XRD analysis (Supplementary Fig. 1 ). TiO 2 nanofibers showed intensive reflections belonging to anatase (JCPDS No. 21-1272) and rutile (JCPDS No. 21-1276) phases. TC2 showed a similar XRD pattern with pristine TiO 2 , where the reflections of CsPbBr 3 QDs cannot be distinguished due to their low content. Apart from the characteristic reflections of TiO 2 , TC4 showed additional reflections at 21.5° and 30.6°, which corresponded to the (110) and (200) planes of CsPbBr 3 QDs, confirming the formation of TiO 2 /CsPbBr 3 nanohybrids. The morphology and crystalline phase of pristine TiO 2 (Supplementary Fig. 2a ) exhibited a porous nanofibrous shape with an average diameter of 200 nm. The porous feature was further revealed by the N 2 sorption isotherms of TC x (Supplementary Fig. 3 ). All the TC x samples showed similar pore size distributions with a wide range of 10–20 nm, much larger than the size of CsPbBr 3 QDs (6–9 nm). 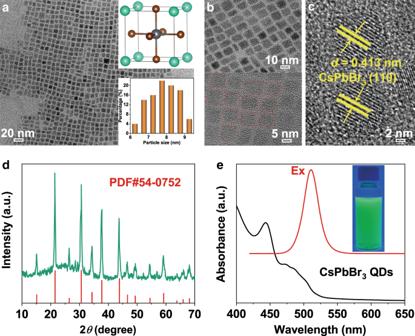Fig. 1: Characterization of CsPbBr3QDs. a,bTransmission electron microscopy (TEM) image and corresponding size distribution (lower right inset of panela), the geometrical structure (upper right inset of panela),chigh-resolution TEM (HRTEM) image,dX-ray diffraction (XRD) pattern, andeUV–vis absorption (black line) and PL emission (red line). Inset shows the photograph of CsPbBr3QDs colloidal solutions in hexane under UV light of 365 nm. The resultant specific surface areas ( S BET ), pore volumes ( V p ), and average pore sizes ( d p ) presented a volcano shape with increasing the loading of CsPbBr 3 QDs (Supplementary Table 1 ). At a low QDs loading (<2 wt.%), TC x showed an increased S BET and reached the maximum value at TC2 because the low filling enables QDs to deposit onto the inner wall of TiO 2 mesopores. Such island-like QDs on the inner wall contribute additional specific surface area for the hybrid. When the QDs loading was further increased, QDs would aggregate in TiO 2 mesopores and the island-like distribution vanished, which thereby resulted in a decrease of S BET . The HRTEM image (Supplementary Fig. 2b ) showed clear lattice spacings of 0.352 and 0.325 nm, corresponding to anatase (101) and rutile (110) d-spacings, respectively. After the assembling process, the QDs were uniformly deposited on the TiO 2 nanofibers (Fig. 2a, b ). The lattice spacings of anatase and rutile phase TiO 2 , as well as CsPbBr 3 QDs, appeared in the HRTEM image, as shown in Fig. 2c , confirming the formation of TiO 2 /CsPbBr 3 nanohybrids. The energy-dispersive X-ray spectroscopy (EDX) spectrum of TC2 (Fig. 2d ) revealed the existence of Cs, Pb, and Br apart from the dominant Ti and O elements. All the elemental mappings overlapped perfectly (Fig. 2e ). Fourier-transform infrared (FTIR) spectra showed the presence of (Ti)–OH on TiO 2 and organic residues on QDs (Supplementary Fig. 4a, b ) [32] . The (Ti)–OH signal weakened upon QDs deposition owing to the shielding effect of QDs. All the results confirmed the successful electrostatic assembly of TiO 2 nanofibers and CsPbBr 3 QDs. Fig. 2: Morphology and structure of TiO 2 /CsPbBr 3 heterojunction. a – c Transmission electron microscopy (TEM), STEM, and high-resolution TEM (HRTEM) images of TC2, d EDX spectrum of TC2, and e high-angle annular dark-field (HAADF) image and EDX elemental mappings of Ti, O, Cs, Pb, and Br elements in TC2. Full size image The optical absorption of the samples was investigated by UV–vis diffuse reflectance spectrometer (DRS) (Supplementary Fig. 5a ). The absorption edges of pristine TiO 2 nanofibers and CsPbBr 3 QDs were located at 400 and 550 nm, corresponding to the bandgap energy of 3.10 and 2.24 eV, respectively (Supplementary Fig. 5b ). In comparison with pristine TiO 2 , TC x showed two obvious absorption edges belonging to TiO 2 and CsPbBr 3 QDs, and exhibited slightly enhanced UV and visible-light harvesting when increasing the amount of CsPbBr 3 QDs owing to the strong light-harvesting capability of perovskite QDs. Note that the calculated bandgap energy of TiO 2 and CsPbBr 3 in TC4 was different from their intrinsic bandgap, implying that there exist electrostatic attraction and interaction between TiO 2 and CsPbBr 3 during the hybridization. X-ray photoelectron spectroscopy (XPS) was further performed to explore the chemical states of the resultant samples. The survey XPS spectrum (Supplementary Fig. 6a ) showed the presence of Cs, Pb, and Br elements within TC2, as well as Ti and O. The ex-situ Ti 2 p XPS spectra of TiO 2 and TC2 (Fig. 3a ) showed symmetrical Ti 2 p doublets of Ti 4+ ions. The O 1 s XPS spectra (Fig. 3b ) revealed the presence of lattice oxygen (529.3 eV) and –OH surface group (531.2 eV). Interestingly, TC2 showed a weaker XPS signal of –OH than pristine TiO 2 , which was also attributed to an increase of QDs over TiO 2 nanofiber surface and was in agreement with the above FTIR results. The Br 3 d -binding energies (BEs) of CsPbBr 3 QDs were 67.8 and 69.8 eV, corresponding to Br 3 d 5/2 and Br 3 d 3/2 , respectively (Fig. 3c ). Noticeably, the BEs of Ti 2 p and O 1 s in TC2 were shifted by 0.2 eV toward a lower BE in comparison with those of pristine TiO 2 , while the Cs 3 d , Pb 4 f (Supplementary Fig. 6c, d ) and Br 3 d BEs of TC2 became more positive as compared with those of QDs, indicating that the electrons transferred from CsPbBr 3 QDs to TiO 2 upon hybridization due to the difference of their work functions. Such electron transfer created an IEF at interfaces pointing from QDs to TiO 2 , facilitating the construction of S-scheme TiO 2 /CsPbBr 3 heterojunction without any redox mediator, which would efficiently separate the charge carriers and thus promote the CO 2 photoreduction [33] , [34] , [35] . Fig. 3: Electron transfer between TiO 2 and CsPbBr 3 quantum dots (QDs). In-situ and ex-situ X-ray photoelectron spectroscopy (XPS) spectra of a Ti 2 p , b O 1 s , and c Br 3 d of TiO 2 , CsPbBr 3 , and TC2. In-situ XPS spectra were collected under UV–vis light irradiation. The electrostatic potentials of d anatase TiO 2 (101), e rutile TiO 2 (110), and f CsPbBr 3 (001) facets. The blue, red, green, gray, and brown spheres stand for Ti, O, Cs, Pb, and Br atoms, respectively. Blue and red dashed lines indicate the Fermi and vacuum energy levels. Full size image Work function ( Φ ), as another important parameter to study the electron transfer within duplicate semiconductor heterostructures, can be estimated from the energy difference of vacuum and Fermi levels according to the electrostatic potential of a material. As shown in Fig. 3d–f , the work function of anatase TiO 2 (101), rutile TiO 2 (110), and CsPbBr 3 QDs (001) were 7.18, 7.08, and 5.79 eV, respectively, indicating that both anatase and rutile TiO 2 have lower Fermi levels than CsPbBr 3 QDs. When they contacted with each other, electrons would flow from CsPbBr 3 to anatase and/or rutile TiO 2 to enable the phases at the same Fermi level and definitely created an IEF at TiO 2 /CsPbBr 3 interfaces. These results were absolutely consistent with above ex-situ XPS results and beneficial to the charge separation and CO 2 photoreduction activity. CO 2 photoreduction activity of TiO 2 /CsPbBr 3 hybrids The CO 2 photoreduction activity of resultant samples was measured in a closed gas-circulation system (Supplementary Fig. 7 ) with a Quartz and Pyrex glass hybrid reaction cell (Supplementary Fig. 8 ) and the photocatalytic reduction products consisted of a majority of CO and a small amount of H 2 . The original chromatograms for the reduction of CO 2 on sample TC2 are shown in Supplementary Fig. 9 . Control experiments (Supplementary Fig. 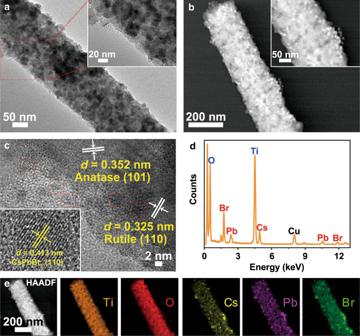Fig. 2: Morphology and structure of TiO2/CsPbBr3heterojunction. a–cTransmission electron microscopy (TEM), STEM, and high-resolution TEM (HRTEM) images of TC2,dEDX spectrum of TC2, andehigh-angle annular dark-field (HAADF) image and EDX elemental mappings of Ti, O, Cs, Pb, and Br elements in TC2. 10 and Table 2 ) showed that neither H 2 nor CO was detected in the dark or in the absence of CO 2 , suggesting that the light irradiation and input CO 2 were indispensable for the photocatalytic reaction. As shown in Fig. 4a, b , pristine TiO 2 and CsPbBr 3 QDs exhibited relatively lower production rates of H 2 (0.12 and 0.06 μmol g –1 h –1 , respectively) and CO (4.68 and 4.94 μmol g –1 h –1 , respectively), resulting from the rapid charge recombination. Note that the H 2 and CO productions were greatly enhanced with increased loading of QDs, and the generation of CO reached a maximum rate (9.02 μmol g –1 h –1 ) with a relatively high selectivity (95%) over TC2, due to the efficient charge separation of TiO 2 /CsPbBr 3 heterostructure. Further increasing CsPbBr 3 QDs amount would be detrimental to the photocatalytic activity (e.g., TC3 and TC4), because the overloading of CsPbBr 3 could shield the light absorption of TiO 2 and decrease S BET of the nanohybrids. Interestingly, with the reaction time went on, the amount of O 2 decreased first and then increased, as shown in Fig. 4c . The initial O 2 in the system came from the input high-purity CO 2 . In the first two hours of photocatalytic CO 2 reduction, the fresh materials exhibit relatively strong reactivity of photoreduction. As a competitive reaction to CO 2 reduction, the consumption rate of O 2 (O 2 + e – → ·O 2 – ) was much higher than the production rate at the initial 2 h, while in the following 2 h, the production rate of O 2 was higher than the consumption rate, the total amount of oxygen and the ratio of oxygen:nitrogen have increased to a certain extent. Fig. 4: CO 2 photoreduction performance and the photocatalytic mechanism of S-scheme heterojunction. Photocatalytic activities of CO 2 reduction over TiO 2 , TC x , and CsPbBr 3 quantum dots (QDs) during 4-h experiment performed under UV–vis light irradiation: time course of a H 2 , b CO, and c O 2 production yields. The initial O 2 concentrations were normalized. d Mass spectra of 13 CO and total ion chromatography (inset) over TC2 in the photocatalytic reduction of 13 CO 2 . Optimized structures of CO 2 molecule adsorbed on e anatase TiO 2 (101), f rutile TiO 2 (110), and g CsPbBr 3 (001) facets. The blue, red, green, gray, and brown spheres stand for Ti, O, Cs, Pb, and Br atoms, respectively. h The DOS of CsPbBr 3 . i Schematic illustration of TiO 2 /CsPbBr 3 heterojunction: internal electric field (IEF)-induced charge transfer, separation, and the formation of S-scheme heterojunction under UV–visible-light irradiation for CO 2 photoreduction. j Time-resolved photoluminescence (TRPL) spectra of TiO 2 (T) and TC2 at emission wavelengths of 450 and 520 nm, respectively. Full size image The recyclability and stability of TC2 for CO 2 photoreduction were investigated (Supplementary Fig. 11 ). After four times cycles, the decay of photocatalytic production yields of H 2 and CO were hardly perceptible. To evaluate the photostability of the nanohybrids, we have characterized the recycled photocatalyst using XRD, TEM, XPS, and FTIR. As shown in the XRD pattern (Supplementary Fig. 12a ), the used photocatalyst showed no detectable phase change. The TEM image confirms that the QDs did not show obvious aggregation after cycled photocatalytic reactions, and the morphology was well maintained (Supplementary Fig. 12b ). The chemical states of the used photocatalyst were also consistent with those of the fresh one, as examined by XPS (Supplementary Fig. 13 ). The FTIR spectra of TC2 before and after reaction were presented in Supplementary Fig. 14 . The characteristic absorbance bands of the aliphatic species from QDs showed no obvious variation, implying that the capping agent of QDs was stable and was not decomposed during the photocatalytic CO 2 reduction. To determine the origin of CO 2 photoreduction products, we performed an isotope-labeled carbon dioxide ( 13 CO 2 ) photocatalytic reduction over TC2. Since the amount of products without photosensitizer and hole sacrificial agent was beyond the detection limit of mass spectrometry detector, we added tris(2,2’-bipyridyl)ruthenium(II) chloride hexahydrate ([Ru II (bpy) 3 ]Cl 2 ·6H 2 O) [36] and 1,3-dimethyl-2-phenyl-2,3-dihydro-1H-benzo[d]imidazole (BIH) [37] into the system to promote the photocatalytic activity, which behaved as the photosensitizer and hole sacrificial agent, respectively. In this case, the production yields of H 2 and CO were significantly enhanced (Supplementary Fig. 15 and Table 2 ) and readily detected by gas chromatography–mass spectrometer (GC-MS). As shown in Fig. 4d , the total ion chromatographic peak ~3.44 min corresponded to CO, which produced three signals in the mass spectra. The main MS signal at m/z = 29 belonged to 13 CO and the others ( 13 C at m/z = 13 and O at m/z = 16) corresponded to the fragments of 13 CO, confirming that the CO product exactly originated from the CO 2 photoreduction over TiO 2 /CsPbBr 3 [38] , [39] . In addition, the total ion chromatographic peaks ~2.36 and 2.48 min can be assigned to the O 2 and N 2 , respectively (Supplementary Fig. 16 ). The CO 2 adsorption of a photocatalyst is an essential step for CO 2 photoreduction [40] . Figure 4e–g compared the optimized models of one CO 2 molecule adsorbed on anatase TiO 2 (101), rutile TiO 2 (110), and CsPbBr 3 (001) surfaces. 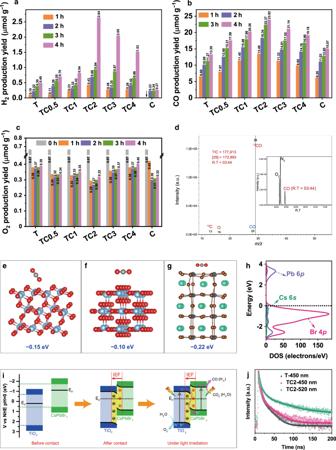Fig. 4: CO2photoreduction performance and the photocatalytic mechanism of S-scheme heterojunction. Photocatalytic activities of CO2reduction over TiO2, TCx, and CsPbBr3quantum dots (QDs) during 4-h experiment performed under UV–vis light irradiation: time course ofaH2,bCO, andcO2production yields. The initial O2concentrations were normalized.dMass spectra of13CO and total ion chromatography (inset) over TC2 in the photocatalytic reduction of13CO2. Optimized structures of CO2molecule adsorbed oneanatase TiO2(101),frutile TiO2(110), andgCsPbBr3(001) facets. The blue, red, green, gray, and brown spheres stand for Ti, O, Cs, Pb, and Br atoms, respectively.hThe DOS of CsPbBr3.iSchematic illustration of TiO2/CsPbBr3heterojunction: internal electric field (IEF)-induced charge transfer, separation, and the formation of S-scheme heterojunction under UV–visible-light irradiation for CO2photoreduction.jTime-resolved photoluminescence (TRPL) spectra of TiO2(T) and TC2 at emission wavelengths of 450 and 520 nm, respectively. Clearly, the adsorption energy ( E ads ) of CO 2 onto CsPbBr 3 (−0.22 eV) was more negative than that onto anatase and rutile TiO 2 (−0.15 and −0.10 eV), which suggests that CO 2 molecules adsorbed on CsPbBr 3 is more stable than on TiO 2 . The results also indicate that CsPbBr 3 QDs were in favor of the adsorption of CO 2 molecules and the photocatalytic CO 2 reduction. To further explore the photocatalytic mechanism, the band structures of TiO 2 and CsPbBr 3 QDs were investigated. The valence band (VB) potential was obtained by analyzing the VB XPS spectra. As shown in Supplementary Fig. 17a, b , the energy level of valence band maximum (VBM) of TiO 2 and CsPbBr 3 is 2.39 and 1.03 eV, respectively. Mott–Schottky (M–S) curves showed that TiO 2 and CsPbBr 3 were of n-type semiconductors and had flat-band potentials of 0.01 eV and −0.51 eV (vs. NHE), respectively (Supplementary Fig. 17c, d ). Thus, the band structures of TiO 2 and CsPbBr 3 QDs can be derived, and the positions of VBM and conduction band minimum (CBM) of TiO 2 and CsPbBr 3 are shown in Supplementary Fig. 17f . Photocatalytic mechanism of S-scheme heterojunction From the above analysis, the superior photoreduction activity was ascribed to the stronger CO 2 adsorption of CsPbBr 3 QDs and the formation of S-scheme heterojunction between TiO 2 and CsPbBr 3 QDs. As revealed by the above ex-situ XPS and DFT analyses, TiO 2 has a lower Fermi level than CsPbBr 3 QDs before they contact. Upon hybridization, the electrons preferred to flow from CsPbBr 3 QDs to TiO 2 , which created an IEF at TiO 2 /CsPbBr 3 interfaces pointing from CsPbBr 3 to TiO 2 and bent the energy bands of TiO 2 and CsPbBr 3 . Upon photoexcitation, the VB electrons of TiO 2 and CsPbBr 3 jumped to their CBs. Driven by the interfacial IEF and bent bands, the photogenerated electrons in TiO 2 CB spontaneously slid toward CsPbBr 3 and recombined with the holes in CsPbBr 3 VB. The electron-rich CsPbBr 3 QDs then acted as active sites and donated electrons to activated CO 2 molecules for producing H 2 and CO. Noted that Pb was the active site for CO 2 photoreduction since the CB of CsPbBr 3 was mainly consisted of Pb 6 p orbitals as evidenced by the density of states (DOS) of CsPbBr 3 (Fig. 4h ). Clearly, the transportation of photoinduced charge carriers follows a slide-like pathway, which implies the presence of S-scheme heterojunction between TiO 2 and CsPbBr 3 QDs. This unique S-scheme charge transfer efficiently separated the photoinduced electron–hole pairs and meanwhile remained the high redox ability of electrons in CsPbBr 3 CB and holes in TiO 2 VB, respectively. The S-scheme heterostructure of TiO 2 /CsPbBr 3 QDs along with the charge transfer and separation is illustrated in Fig. 4i . Such an S-scheme charge transfer route was strongly evidenced by the in-situ XPS spectra measured under light irradiation. As revealed in Fig. 3a–c and Supplementary Fig. 6c, d , the BEs of Ti 2 p and O 1 s for TC2 under light irradiation shifted positively by 0.3 eV with reference to those in the corresponding ex-situ spectra. Conversely, the BEs of Cs 3 d , Pb 4 f , and Br 3 d of TC2 shifted negatively by 0.5 eV. The BE shifts unequivocally proved that the photoexcited electrons in TiO 2 CB transferred to CsPbBr 3 QDs VB under light irradiation, following an S-scheme pathway, which supported the proposed photocatalytic mechanism. It is worth mentioning that the TiO 2 we used consisted of both anatase and rutile phases, and the charge transfer between the two phases may take place as a result of forming homojunction. As evidenced by DFT results (Fig. 3d, e ), the work function of anatase TiO 2 (101) was larger than that of rutile TiO 2 (110), indicating that electrons would flow from rutile to anatase and created an IEF at anatase/rutile TiO 2 interfaces. Driven by the interfacial IEF, the photogenerated electrons in anatase TiO 2 CB spontaneously slid toward rutile TiO 2 VB and recombined with the holes in the rutile TiO 2 VB. Such transportation of photoinduced charge carriers follows an S-like pathway (S-scheme homojunction) between anatase and rutile TiO 2 (Supplementary Fig. 18 ), which is consistent with our previous work [41] . When CsPbBr 3 QDs deposited on TiO 2 nanofibers, all possible schematic illustrations between anatase TiO 2 , rutile TiO 2 , and CsPbBr 3 QDs are shown in Supplementary Fig. 19 . To further prove the efficient charge separation of TiO 2 /CsPbBr 3 S-scheme heterojunction, photoluminescence (PL) emission spectra of the samples were collected (Supplementary Fig. 20 ). TC2 and TC4 showed a marginally lower PL intensity than TiO 2 , implying that the presence of CsPbBr 3 QDs efficiently retarded the electron–hole recombination in TiO 2 . To gain a deeper insight into the charge transfer dynamics, the time-resolved photoluminescence (TRPL) spectra of TiO 2 and TC2 were recorded at emission wavelengths ( E W ) of 450 nm and 520 nm (Fig. 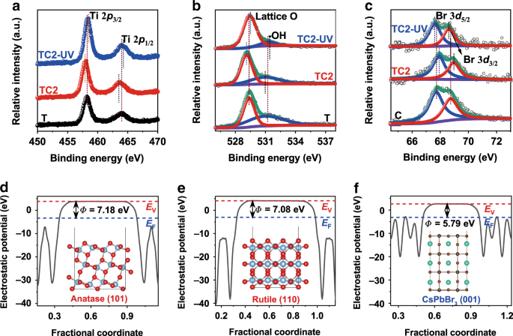4j ), corresponding to the maximum fluorescence emissions of TiO 2 and QDs, respectively. Fig. 3: Electron transfer between TiO2and CsPbBr3quantum dots (QDs). In-situ and ex-situ X-ray photoelectron spectroscopy (XPS) spectra ofaTi 2p,bO 1s, andcBr 3dof TiO2, CsPbBr3, and TC2. In-situ XPS spectra were collected under UV–vis light irradiation. The electrostatic potentials ofdanatase TiO2(101),erutile TiO2(110), andfCsPbBr3(001) facets. The blue, red, green, gray, and brown spheres stand for Ti, O, Cs, Pb, and Br atoms, respectively. Blue and red dashed lines indicate the Fermi and vacuum energy levels. The fitted decay curves disclose the lifetime ( τ ) and percentage ( Rel .%) of charge carriers (Supplementary Table 3 ). The short lifetime ( τ 1 ) corresponds to radiative recombination of the carriers (denoted as τ 1 -carriers), while the long lifetimes ( τ 2 and τ 3 ) correspond to non-radiative recombination and energy-transfer process [42] . Note that the un-recombined τ 1 -carriers will participate in surface photocatalytic reaction. Thus, the decrease of τ 1 -carrier percentage implies radiative recombination inhibited. At E W = 450 nm, only TiO 2 showed a fluorescence emission signal. As shown in Supplementary Table 3 , TC2 had a lower percentage (36.27%, 450 nm) of τ 1 -carriers than pristine TiO 2 (37.98%, 450 nm), suggesting the radiative recombination over TiO 2 was inhibited upon QDs deposition due to the formation of S-scheme heterojunction [43] , [44] . Further, a similar decrease in τ 1 -carrier percentage was also observed at E W = 520 nm. Notably, TC2 showed longer lifetime than pristine TiO 2 due to the transfer of the electrons in TiO 2 CB to QDs VB. Therefore, it is not surprising that the TC2 composite sample exhibited enhanced photocatalytic CO 2 reduction performance. The electrochemical impedance spectra (EIS) (Supplementary Fig. 21a ) showed the samples with CsPbBr 3 QDs exhibited smaller semicircle compared to pure TiO 2 and revealed lower charge-transfer resistance. The polarization curves of TiO 2 and TC2 under light irradiation (Supplementary Fig. 21b ) showed that the overpotential for TC2 was much lower than that of TiO 2 , indicating that TiO 2 /CsPbBr 3 hybrids presented better reduction capability than that of TiO 2 . These results proved that CsPbBr 3 QDs, as an emerging semiconductor, could form S-scheme heterojunction with TiO 2 to promote the electron transfer and separate the electron–hole pairs for efficient CO 2 photoreduction. In summary, an S-scheme TiO 2 /CsPbBr 3 heterojunction synthesizes through an electrostatic assembly method. The resulting TiO 2 /CsPbBr 3 heterojunction reveals an enhanced activity toward CO 2 photoreduction under UV–visible-light irradiation due to the IEF-induced, more efficient charge separation between TiO 2 and CsPbBr 3 . DFT calculations reveal the work function of TiO 2 was greater than that of CsPbBr 3 , implying electrons transfer from CsPbBr 3 to TiO 2 upon hybridization and thus created an IEF at interfaces. The IEF drives photoinduced electrons in TiO 2 CB to immigrate to CsPbBr 3 VB as evidenced by in-situ XPS analysis, confirming an S-path of charge transfer. Isotope ( 13 CO 2 ) tracer results confirm that the reduction products originate from CO 2 source, instead of any contaminant carbon species. This work provides a point of view in the design of photocatalysts with distinct heterojunctions for efficient photocatalytic CO 2 reduction. Synthesis of electrospun TiO 2 nanofibers All the chemicals were of analytic grade and purchased from Shanghai Chemical Company. Typically, tetrabutyl titanate (TBT, 2.0 g) and poly(vinyl pyrrolidone) (PVP, 0.75 g, MW = 1,300,000) were mixed with ethanol (10.0 g) and acetic acid (2.0 g) to form a transparent pale-yellow solution after magnetic stirring for 5 h. Afterward, the solution was transferred into a 10-mL syringe in an electrospinning setup with a voltage of 20 kV and a solution feeding rate of 2.5 mL h –1 . The needle-to-collector distance was 10 cm. The collected TiO 2 precursor was annealed at 550 °C for 2 h with a heating rate of 2 °C min –1 in air. Synthesis of perovskite CsPbBr 3 QDs Briefly, 130 mg of Cs 2 CO 3 (0.4 mmol) were mixed with octadecylene (ODE, 6 mL) and oleic acid (OA, 0.5 mL) under stirring in a three-neck flask (25 mL). The mixture was dried at 120 °C for 1 h under vacuum and heated to 150 °C under N 2 gas to form Cs(oleate) solution, which was stored at room temperature and preheated to 140 °C prior to use. Then 72 mg of PbBr 2 (0.196 mmol) was mixed with ODE (5.0 mL), oleylamine (0.5 mL), and OA (0.5 mL) in another flask (25 mL), and was dried under vacuum at 105 °C for 0.5 h. The mixture was heated to 170 °C, and Cs(oleate) (0.45 mL) was rapidly injected under vigorously stirring for 5 s. The reaction was quenched by immersing the flask into an ice-water bath. The obtained product was mixed with 3 mL of hexane and centrifuged at 1208 × g for 2 min to remove aggregates and large particles. The supernatant was precipitated with acetone and centrifuged at 3355 × g for 5 min. As-collected CsPbBr 3 QDs were re-dispersed in hexane for further use. Preparation of TiO 2 /CsPbBr 3 heterostructures Typically, 200 mg of TiO 2 nanofibers were dispersed into 20 mL of hexane. A certain amount of CsPbBr 3 QDs solution was added into TiO 2 suspension under vigorous stirring for 2 h. TiO 2 and CsPbBr 3 QDs were assembled by electrostatic self-assembly. The mixture was then vacuum-dried at 50 °C for 2 h to form TiO 2 /CsPbBr 3 heterostructures. The products are labeled as TC x , where T and C denote TiO 2 and CsPbBr 3 QDs, respectively; x is the mass percentage of CsPbBr 3 QDs. Characterization XRD was performed on a D/Max-RB X-ray diffractometer (Rigaku, Japan) with Cu Kα radiation. TEM images were observed on a Titan G2 60-300 electron microscope equipped with an EDX spectrometer. UV–visible DRS was collected on a Shimadzu UV-2600 UV–visible spectrophotometer (Japan). XPS was performed on a Thermo ESCALAB 250Xi instrument with Al K α X-ray radiation. In-situ XPS was conducted under the same condition, except that UV–visible-light irradiation was introduced. FTIR spectra were recorded with an attenuated total reflectance (ATR) mode on Nicolet iS 50 (Thermo Fisher, USA). The PL emission spectra were collected on a fluorescence spectrophotometer (F-7000, Hitachi, Japan). TRPL spectra were recorded on a fluorescence lifetime spectrophotometer (FLS 1000, Edinburgh, UK) at an excitation wavelength of 325 nm. Electrochemical measurements were conducted on an electrochemical analyzer (CHI660C, CH Instruments, Shanghai). Pt wire, Ag/AgCl (saturated KCl), and 0.5 M Na 2 SO 4 solution functioned as the counter electrode, reference electrode, and electrolyte, respectively. For the working electrode, 20 mg of TC x was ground in 1.0 mL of ethanol and 10 μL of Nafion solution to make a slurry, which was coated onto F-doped SnO 2 -coated (FTO) glass with an exposed area of 1 cm 2 . The FTO electrode was then vacuum-dried at 60 °C for 1 h. Photocatalytic CO 2 reduction The photocatalytic CO 2 reduction was performed in a gas-closed system equipped with a gas-circulated pump. The apparatus of the system is shown in Supplementary Fig. 7 . Typically, 10 mg of photocatalysts, 30 mL of acetonitrile, and 100 μL of water were added in a Quartz and Pyrex glass hybrid reaction cell (Supplementary Fig. 8 ). The airtight system was completely evacuated by using a vacuum pump. Then ~80 kPa of high-purity CO 2 (99.999%) gas was injected. After adsorption equilibrium, the photocatalytic cell was irradiated with a 300 W Xe arc lamp (PLS-SXE300D, Beijing Perfectlight, China), and the reaction system was kept at 10 °C as controlled by cooling water. The CO 2 -reduction products were analyzed on a gas chromatograph (GC-2030, Shimadzu Corp., Japan) equipped with a barrier discharge ionization detector (BID) and a capillary column (Carboxen 1010 PLOT Capillary, 60 m × 0.53 mm). The column was maintained at 35 °C for 15 min. It was then heated to 180 °C at 20 °C min –1 , and maintained for another 5 min. Helium was the carrier gas with pressure set to 70 kPa. The temperatures of the injector and BID were set to be 150 and 280 °C, respectively. For comparison, 2 mM of tris(2,2′-bipyridyl)ruthenium(II) chloride hexahydrate ([Ru II (bpy) 3 ]Cl 2 ·6H 2 O) and 10 mM of 1,3-dimethyl-2-phenyl-2,3-dihydro-1H-benzo[d]imidazole (BIH) were added into the photocatalytic system (other parameters were unchanged), which behaved as the photosensitizer and hole sacrificial agent, respectively. A series of control experiments were also conducted, and the results are summarized in Supplementary Table 2 . Isotope-labeling measurement The isotope-labeling experiment was conducted by using 13 CO 2 (isotope purity, 99% and chemical purity, 99.9%, Tokyo Gas Chemicals Co., Ltd.) as the carbon source. Typically, 10 mg of photocatalysts, 2 mM of [Ru II (bpy) 3 ]Cl 2 ·6H 2 O, 10 mM of BIH, 30 mL of acetonitrile and 100 μL of water were loaded into the reaction cell. The protocol of 13 CO 2 photoreduction was the same as that mentioned above. The gas products were analyzed by gas chromatography–mass spectrometry (JMS-K9, JEOL-GCQMS, Japan and 6890 N Network GC system, Agilent Technologies, USA) equipped with the column for detecting the products of 13 CO (HP-MOLESIEVE, 30 m × 0.32 mm × 25 μm). Helium was used as carrier gas. The column was maintained at 60 °C for 20 min, and the flow of the carrier was 0.5 ml L –1 . The temperatures of the injector, EI source, and the GCITF were set to be 200, 200, and 250 °C, respectively.